Self-propagating high-temperature synthesis for compound thermoelectrics and new criterion for combustion processing The existing methods of synthesis of thermoelectric (TE) materials remain constrained to multi-step processes that are time and energy intensive. Here we demonstrate that essentially all compound thermoelectrics can be synthesized in a single-phase form at a minimal cost and on the timescale of seconds using a combustion process called self-propagating high-temperature synthesis. We illustrate this method on Cu 2 Se and summarize key reaction parameters for other materials. We propose a new empirically based criterion for sustainability of the combustion reaction, where the adiabatic temperature that represents the maximum temperature to which the reacting compact is raised as the combustion wave passes through, must be high enough to melt the lower melting point component. Our work opens a new avenue for ultra-fast, low-cost, large-scale production of TE materials, and provides new insights into combustion process, which greatly broaden the scope of materials that can be successfully synthesized by this technique. Thermoelectric (TE) materials convert heat into electricity directly through the Seebeck effect or operate as heat pumps using the Peltier effect. TE energy conversion has drawn much attention to applications in areas such as solar thermal conversion [1] , industrial waste heat recovery [2] , spot cooling of electronic devices [3] and air conditioning [4] . The efficiency of a TE material is judged by its dimensionless figure of merit ZT , defined as ZT = α 2 σT / κ , where α , σ , κ and T are the Seebeck coefficient, electrical conductivity, total thermal conductivity and the absolute temperature, respectively. To achieve high conversion efficiency, a large ZT is required. High electrical conductivity (corresponding to low Joule heating), large Seebeck coefficient (corresponding to a large potential difference) and low thermal conductivity (supporting a large temperature difference) are the necessary attributes of an efficient TE material. However, the above three transport parameters are strongly interdependent and thus it is a challenging task to optimize the TE figure of merit. Most existing studies have focused on the optimization of TE properties by appropriate doping and on minimizing the thermal conductivity by enhancing phonon scattering by a variety of means [5] , [6] , [7] , [8] , [9] , [10] , [11] , [12] , [13] , [14] , [15] , [16] , [17] , [18] , [19] , [20] , [21] . Among the most successful approaches has been the introduction of finely dispersed nanoinclusions, particularly if such nanoinclusions are coherent (endotaxial) with the matrix material and thus have a minimal negative impact on the charge carrier transport [7] , [8] , [9] , [10] , [11] , [12] , [13] , [14] , [15] . Efficient synthesis and its adaptability to a large-scale industrial processing are important issues determining the economic viability of the fabrication process. So far, TE materials have been synthesized mostly by one of the following methods: melting followed by slow cooling [9] ; melting followed by long time annealing [20] , multi-step solid-state reactions [16] and mechanical alloying [17] . Each such processing is time and energy consuming and not always easily scalable. Moreover, it is often very difficult to control the desired stoichiometry and microstructure. An interesting alternative method for synthesizing compounds is the combustion synthesis, which relies on exothermic reactions. The combustion synthesis is exceptionally fast, typically on the timescale of seconds and its important feature is a precise control of composition. The technique has been originally developed and used in the synthesis of refractory materials [22] , high purity ceramics [23] and intermetallics [24] . The combustion synthesis process is subdivided into two distinct modes of ignition. The first is termed thermal explosion, in which the whole volume of the compact is heated to the ignition temperature at which all reactant constituents spontaneously react to a final product. This technique has been used for the synthesis of a few TE materials [25] but the purity of the final product is hard to control and multiple phases are often present. The second ignition mode is self-propagating high-temperature synthesis (SHS) in which the synthesis is initiated by point-heating a small part (usually the top) of the sample. Once started, a wave of exothermic reactions (combustion wave) passes through the remaining material as the liberated heat of fusion in one section is sufficient to maintain the reaction in the neighbouring section of the compact. As the combustion wave passes through the sample it purifies the material and maintains its stoichiometry. Current understanding of the process requires achieving sufficiently high adiabatic temperature ( T ad ≥1,800 K) that represents the maximum temperature to which the reacting compact is raised as the combustion wave passes through [26] , [27] , [28] . This technique has been tried recently with oxide thermoelectrics [29] , [30] but resulted in a multiphase material. The appealing attributes of the SHS synthesis, namely its fast one-step process requiring minimum of energy and its scalable nature, together with the fact that the final product maintains the desired stoichiometry, provided enough temptation and curiosity for us to try to apply it to a wide range of TE materials including Cu 2 Se. Faced with a highly restrictive criterion imposed on the adiabatic temperature ( T ad ≥1,800 K), we were concerned that the SHS synthesis would not be feasible because of the very high temperature of 1,800 K at which most TE compounds would decompose due to high volatility of constituent elements. To our great surprise, the SHS works and the reaction takes place at temperatures considerably lower than what the literature data indicated. Here we report a successful synthesis of single-phase TE materials by SHS. We provide a detailed account of reaction parameters and transport properties of Cu 2 Se and, in a tabular form, summarize data on all other TE materials we synthesize by this process. We also offer a new empirically based criterion for the applicability of the SHS process that greatly expands the range of materials that can be synthesized by this technique. The spectacular success of being able to synthesize compound thermoelectrics in their single phase by SHS bodes well for economical fabrication of efficient TE materials. 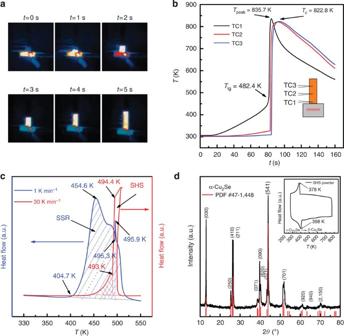Figure 1: Characteristics of the SHS synthesis. (a) Infrared photos of different stages of the SHS process. (b) Temperature profile of thermocouples at different positions. (c) DSC curves of the SHS process. (d) XRD pattern of the SHS product, the inset shows DSC cycling of the SHS product. SHS synthesis of Cu 2 Se Figure 1a shows infrared images of Cu 2 Se in three different stages of the SHS process: (i) local ignition; (ii) combustion wave passing through and (iii) product cooling. As already mentioned, the entire process takes a few seconds. We record temperature changes as the combustion wave passes by different positions along the length of a rectangular-shaped pellet. For illustration purpose, the pellet is in air, however, in the actual synthesis, pellets are sealed in a silica tube under vacuum. In both cases, the synthesized product is a single-phase material, as shown in Supplementary Fig. 1 . Figure 1b shows the temperature profile of the SHS reaction as recorded by thermocouples TC1–TC3 located in positions shown in the inset of Fig. 1b . The initial heating rate obtained from the temperature profile in Fig. 1b is >200 K s −1 . The maximum temperature reached in the centre of the pellet is 835 K. After reaching the maximum temperature, the pellet cools down rapidly. The speed of propagation of the combustion front, 5.6 mm s −1 , is calculated by dividing the distance between the thermocouples by the time difference at which the thermocouples reach a certain temperature. The resulting speed is rather low but within the range of 1–250 mm s −1 reported in the literature for combustion fronts in other SHS-processed materials [26] , [27] , [28] , [31] . Figure 1c shows differential scanning calorimetry (DSC) curves for the mixture of Cu and Se powders with the intended stoichiometry of Cu 2 Se corresponding to two very different heating rates. When the DSC operates with the heating rate of 1 K min −1 , the exothermic peak is quite wide and the heat flow rate is low, a situation corresponding to solid-state reaction processing. In contrast, when the heating rate is increased to 30 K min −1 , the exothermic peak becomes sharp and huge. Figure 1d shows the x-ray diffraction (XRD) pattern of the reacted material after SHS. The data demonstrate that the reacted material is a single-phase α-Cu 2 Se structure in accord with JSPDS47-1448. The inset of Fig. 1d shows the DSC curve of the material after SHS. A characteristic feature of Cu 2 Se—the reversible α–β phase transition taking place at about 398 K—is clearly revealed. The back-scattered electron image, wavelength-dispersive x-ray spectroscopy and electron-probe micro-analysis (EPMA) indicate that the reacted product after SHS is a perfectly homogeneous chemical compound without the presence of any obvious secondary phase. The actual composition of the reacted material measured at several different locations is Cu 2.004 Se, consistent with the nominal composition. Thus, SHS processing controls the composition very precisely and yields homogeneous Cu 2 Se in a time span of few seconds. A more detailed description of the mechanism precisely controlling the composition and images of the resulting microstructure are available in Supplementary Figs 2–4 . Supplementary Movies of the SHS processing are also provided. Figure 1: Characteristics of the SHS synthesis. ( a ) Infrared photos of different stages of the SHS process. ( b ) Temperature profile of thermocouples at different positions. ( c ) DSC curves of the SHS process. ( d ) XRD pattern of the SHS product, the inset shows DSC cycling of the SHS product. Full size image The temperature dependence of TE properties of the Cu 2 Se compound is shown in Fig. 2 . To verify the measurements and their reproducibility, we have cross-checked the data with measurements carried out at the University of Michigan on samples cut from the same ingot. Overall, the data agree to within 10%. The sample marked as SHS–spark plasma sintering (SPS)-WH is subsequently annealed at 800 K for 3 weeks and is marked as such. The temperature dependence of the electrical conductivity for the Cu 2 Se compound is shown in Fig. 2a . The electrical conductivity decreases with increasing temperature, displaying a metallic behaviour. The higher electrical conductivity of Cu 2 Se synthesized by SHS–SPS in comparison to the M-AN-SPS sample [32] is ascribed to its higher carrier concentration. All transport data show a discontinuity near 396 K associated with the α–β phase transition [33] . The temperature dependence of the Seebeck coefficient of Cu 2 Se compounds is shown in Fig. 2b . In the entire temperature range the Seebeck coefficient is positive in accord with the behaviour of the Hall effect as shown in Supplementary Table 1 . The Seebeck coefficient increases with the increasing temperature and reaches values in excess of 230 μV K −1 at 1,000 K. This value is somewhat lower than the value measured on the M-AN-SPS sample, consistent with the higher carrier concentration of our SHS–SPS sample. However, the power factors of the two samples are comparable. Apparently, the mostly coherent nature of the nanostructure (see Supplementary Fig. 4 ) in SHS–SPS samples has no detrimental impact on the carrier transport. The temperature dependence of the thermal conductivity of Cu 2 Se is shown in Fig. 2c . With the increasing temperature, the thermal conductivity decreases and reaches a low value of 0.65 W m −1 K −1 near 1,000 K. The lower thermal conductivity of the SHS–SPS sample is likely due to enhanced phonon boundary scattering on the nanostructural features (see Supplementary Fig. 4 ) in this sample. 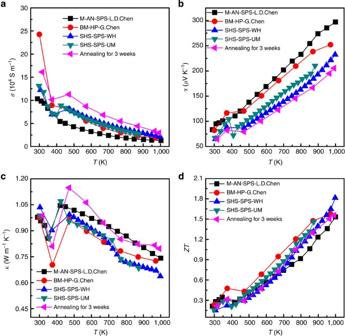Figure 2: Thermoelectric properties of Cu2Se. (a) Temperature-dependent electrical conductivity, (b) Seebeck coefficient, (c) thermal conductivity and (d) thermoelectric figure of the merit of Cu2Se prepared by SHS–SPS. As a result of the low thermal conductivity and excellent electronic properties, the maximum ZT value as high as 1.8 is achieved at 1,000 K. Figure 2: Thermoelectric properties of Cu 2 Se. ( a ) Temperature-dependent electrical conductivity, ( b ) Seebeck coefficient, ( c ) thermal conductivity and ( d ) thermoelectric figure of the merit of Cu 2 Se prepared by SHS–SPS. Full size image An important question pertains to the thermal stability of Cu 2 Se and the reproducibility of its transport properties. It is well-known that the liquid-like nature of Cu in the high-temperature β-phase of the Cu 2 Se structure makes the material thermally unstable at elevated temperatures. To test the stability of our Cu 2 Se prepared by SHS–SPS, we anneal it at 800 K for 3 weeks and re-measured its transport properties. The results are perfectly reproducible and the microstructure, composition and TE properties are unchanged. A detailed account of the stability tests made on a series of SHS–SPS-prepared Cu 2 Se is given in Supplementary Figs 5–7 . While the above test indicates an improved thermal stability of the SHS–SPS sample in comparison to the M-AN-SPS processed sample, it does not address the issue of Cu migration under high current conditions expected during module operation which requires further detailed evaluation. Combustion synthesis of other thermoelectrics Based on the success with the combustion synthesis of Cu 2 Se, we apply the SHS technique to Bi 2 Te 3 , Bi 2 Se 3 , Cu 2 SnSe 3 , ZrNiSn, PbS, PbSe, SnTe, CoSb 3 , Mg 2 Sn and Mg 2 Si. In each case, high purity powders are used as a starting material and weighed according to the desired stoichiometry above. The powders are mixed in an agate mortar and are pressed into pellets. Each respective pellet is sealed in a silica tube under the pressure of 10 −3 Pa. The pellets are locally ignited by the flame of a torch. Supplementary Table 2 shows the thermodynamic data and the corresponding reactions of compounds synthesized by SHS. Parameters related to the combustion synthesis such as the dimension of the pellets, the adiabatic temperature, the method of ignition, the velocity of combustion wave, the ignition temperature and the duration of each combustion reaction are shown in Table 1 . XRD patterns of the powdered samples after combustion synthesis are provided in Supplementary Fig. 8 and Supplementary Note 1 indicate that a single-phase material is obtained for all the above systems within a few seconds. Again, all compounds were synthesized by the combustion synthesis for the first time. It appears that the combustion synthesis is universally applicable to a vast majority of all compound TE semiconductors. It shortens the synthesis time dramatically, and is easily scalable for industrial applications. Having shown that high performance TE Cu 2 Se can be obtained by the SHS method, we then test TE properties of all other compound TE materials prepared by SHS and compare their ZT values with the same materials prepared by traditional synthesis methods. Since the reacted material following the combustion synthesis is rather porous, we powder it and apply SPS to achieve the near theoretical density. In Table 2 we summarize TE properties of such SHS–SPS-prepared compound TE materials. The detailed transport properties are shown in Supplementary Figs 10–14 and Supplementary Note 2 . The figure of merit ZT of samples obtained by SHS–SPS is comparable to or better than samples synthesized by other methods. Thus, the SHS synthesis is exceptional not only from the economic point of view but it actually results in superior TE materials. Table 1 Parameters of SHS for thermoelectric materials. Full size table Table 2 Comparison of thermoelectric properties of samples synthesized by SHS–SPS and by other methods. Full size table New thermodynamic criterion for combustion synthesis Having successfully synthesized many compound TE materials by SHS, we inquire into the conditions necessary for the self-sustaining nature of the combustion process. We notice that once ignited, very high temperatures can be achieved in a short time due to the highly exothermic nature of reactions. It is therefore reasonable to assume that we deal with a thermally isolated exothermic system because there is very little time for the heat to disperse to the surroundings. Therefore, the maximum temperature to which the product is raised can be assumed to be the adiabatic temperature, T ad . In the past, this temperature was considered a key point in evaluating whether the reaction will or will not be self sustaining. Moreover, the morphology and the formation mechanism are very sensitive to T ad (refs 26 , 27 , 28 , 31 , 34 ). Assessing available experimental data for high-temperature ceramics and intermetallics, Merzhanov [26] , [27] , [28] suggested that the system will not be self sustaining unless T ad reaches at least 1,800 K. The heat released, Δ H 298 , in a chemical reaction such as 2Cu+Se→Cu 2 Se, starting from the room temperature, is readily estimated from where C p is the molar specific heat of the product and the integral includes latent heats of melting, vaporization and phase transitions, if any. Using thermodynamic data for Cu 2 Se (ref. 35 ) and equation (1), the calculated adiabatic temperature for Cu 2 Se turns out to be about 1,084 K. In comparison to the measured combustion temperature (823–836 K), this is a somewhat higher temperature, indicating that the sample is not truly adiabatic under conditions of the measurement and some heat escapes to the surroundings. Nevertheless, the adiabatic temperature of Cu 2 Se is dramatically lower than the minimal adiabatic temperature viewed previously as critical to sustain the self-propagating nature of the reaction. As the data in Table 1 document, the same conclusion is reached for all other compound TE materials tested. Obviously, the criterion T ad ≥1,800 K, often quoted in the literature [26] , [27] , [28] , is not universal and certainly not adequate for small gap semiconductors. In Fig. 3a are plotted adiabatic temperatures T ad (the left axis) and the ratio between the calculated formation energy and the heat capacity (the right axis) of each compound TE material (data of current research), as well as high-temperature refractory and intermetallic materials (values from the literature). The data indicate that the adiabatic temperature of all high-temperature intermetallics (borides, carbides and silicates) is, indeed, >1,800 K. Moreover, the ratio between the formation energy and the heat capacity of these compounds is >2,000 K as suggested by Munir [28] . In contrast, the adiabatic temperature of TE semiconductors is dramatically <1,800 K and their formation energy/heat capacity ratio falls mostly well below 2,000 K. As an example, the well-known and important TE compounds Bi 2 Te 3 and Bi 2 Se 3 have their adiabatic temperature well below 1,000 K. According to the criterion T ad ≥1,800 K, the reaction leading to their formation should not have been self sustaining. Obviously, the criterion fails in the case of compound semiconductors. If so, is there another, more universally applicable criterion? 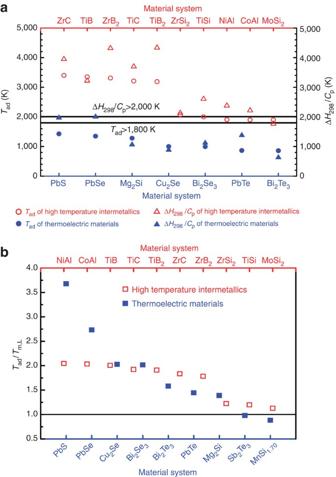Figure 3: New criterion for SHS process. (a) Adiabatic temperatureTadand ΔH298/Cp(298)of materials prepared by SHS. (b) The ratio between the adiabatic temperatureTadand the melting point of the lower melting point componentTm,L. Figure 3: New criterion for SHS process. ( a ) Adiabatic temperature T ad and Δ H 298 / C p(298) of materials prepared by SHS. ( b ) The ratio between the adiabatic temperature T ad and the melting point of the lower melting point component T m,L . Full size image To answer the question, we examine the ratio formed by the relevant thermodynamic parameters: the adiabatic temperature, T ad , divided by the melting temperature of the lower melting point component, T m,L . The ratio T ad /T m,L is displayed in Fig. 3b for both compound thermoelectrics and high-temperature intermetallics, all synthesized by SHS. In this figure, compound TE materials are presented with solid squares, while high-temperature intermetallics are shown with open squares. It follows, based on the available data, that for the SHS reaction to be self sustaining, the value of T ad /T m,L should be >1, that is, the heat released in the reaction must be high enough to melt the component with the lower melting point. When this happens, the higher melting point component rapidly dissolves in the liquid phase of the first component and generates heat at a rate high enough to sustain propagation of the combustion wave. It is interesting to note that, in spite of trying several times, we did not succeed to prepare, by using the SHS synthesis, the two important TE materials, namely Sb 2 Te 3 and MnSi 1.70 (see Supplementary Fig. 9 and Supplementary Note 1 ). Indeed, our attempts have failed because the calculated ratio T ad /T m,L for both materials is less than unity, that is, the heat of reaction is too low to melt the lower melting point component. This impedes the reaction speed and prevents the reaction front to self propagate. Our guideline has a clear physical basis in terms of thermodynamic parameters of the system. Moreover, our new, empirically based criterion covers all existing materials synthesized by SHS whether they are compound TE semiconductors or high-temperature refractory and intermetallic compounds. We show that essentially all compound TE materials can be prepared by a very fast single-step SHS synthesis. This, at a glance, looks very surprising given the existing criterion that requires attaining a minimum adiabatic temperature of some 1,800 K to sustain the propagation of the combustion wave, the essence of this synthesis process. We determine the key synthesis parameters for each of the compound TE materials synthesized by SHS and it is clear that the existing criterion of 1,800 K is entirely inadequate. Based on our empirical data, we are able to formulate a new criterion for the applicability of the SHS synthesis that is based on the thermodynamic parameters of the system. It specifies that the SHS process will proceed whenever the adiabatic temperature exceeds the melting point of the lower melting point component of the compact. The new criterion has a clear physical meaning and covers all existing materials prepared by the SHS synthesis, including high-temperature refractory and intermetallic compounds. Moreover, the new criterion greatly expands the range of materials that can be successfully synthesized by this extraordinarily fast and inexpensive synthesis method. We provide a detailed account of the synthesis and properties of Cu 2 Se, with the parameters of many other compound TE materials presented in a tabular form. The TE performance of samples prepared by SHS is comparable and on many occasions better than materials prepared by the traditional synthetic routes. This research opens the way for ultra-fast, low-cost, mass production fabrication of efficient TE materials based on compound semiconductors. Synthesis and measurements Stoichiometric amounts of high purity Cu (4N) and Se (4N) powders are weighed and mixed in the agate mortar and then cold pressed into a pellet. The pellet is sealed in a silica tube under a pressure of 10 −3 Pa and brought to the ignition point using a torch flame. The propagating combustion wave, see Fig. 1a , reacts Cu and Se inside the silica tube in a time span of few seconds. The reacted pellet is crushed, hand ground into a fine powder and then sintered by SPS at 973 K for 3 min under a pressure of 35 MPa. The structure is characterized by XRD (PANalytical X’Pert Pro X-ray diffraction Cu Kα). The morphology and composition are determined by back-scattered electron imaging (field emission scanning electron microscopy (FESEM); S-8020), energy dispersive x-ray analysis (EDS; Horiba 250), and by EPMA (JXA8800). The microstructure is investigated using transmission electron microscopy (TEM; JEM2100F) with EDS. The electrical conductivity σ and the Seebeck coefficient α are measured simultaneously using a ZEM-3 apparatus. The thermal conductivity κ is calculated from the measured thermal diffusivity D , specific heat C p and density d according to the relationship κ = D × C p × d . The thermal diffusivity and the specific heat are determined using a laser flash method (NETZSCH; LFA 457) and a power-compensation differential scanning calorimeter (TA; DSCQ20), respectively. All measurements are performed in a temperature range of 300–1,000 K. Independent measurements at the UM are carried out using a home-made high-temperature apparatus ( σ and α ) and the ANTER’s Flashline 500 thermal diffusivity apparatus ( D ) in conjunction with the NETZSCH-DSC 404 Pegasus apparatus ( C p ). Mechanism of SHS process To clarify the formation and reaction mechanisms of Cu and Se powders during the processing, a series of DSC and XRD experiments are performed on 20 mg cold-pressed pellets exposed to different temperatures, temperature holding stages and rates of heating. First, the pellet is cycled at temperatures of 413, 433, 453, 473, 493, 513, 533, 553 and 573 K at a rate of 10 K min −1 and held at each temperature for 1 h. From each temperature it is cooled down to 273 K with the cooling rate of 30 K min −1 . All thermal cycling is done under the protection of an Ar gas flowing at a rate of 50 ml min −1 . Supplementary Fig. 2a shows XRD patterns of the pellet after each thermal cycle. The composition evolves but no Cu 2 Se is detected following cycling to temperatures below 493 K. Cycling to temperatures in the range 513–573 K leaves XRD patterns substantially unchanged and the main phase is identified as α-Cu 2−x Se. A small quantity of Cu 1.8 Se and Cu is detected in the XRD pattern, but with the increasing cycling temperature, the signal becomes weaker and weaker and the phase composition approaches the nominal composition. DSC curves show that the α–β phase transition temperature increases with the increasing cycling temperature. The phase transition temperature settles at 399 K after the pellet is cycled to 573 K and held there for 1 h, consistent with the literature value of the α–β phase transition in Cu 2 Se. With the heating rate of 10 K min −1 , the single-phase Cu 2 Se is obtained following cycling to 573 K. To determine the ignition temperature, the pellet is cycled to the same range of temperatures as previously mentioned under the same conditions except that a much faster heating rate of 30 K min −1 is used. As Supplementary Fig. 3 indicates, single-phase Cu 2 Se is obtained following cycling to merely 493 K and even without parking there for 1 h. We have also tried to cycle the pellet to 493 K with a rate of heating of 20 K min −1 , but Cu 2 Se does not form, see Supplementary Fig. 3b . Hence, the ignition temperature is 493 K according to the XRD and DSC results, and for the process to be self sustaining, the heating rate of at least 30 K min −1 is required. The temperature of 493 K is the melting point of Se and thus the ignition point coincides with melting of Se and dissolution of Cu in it. The data indicate that the reaction mechanism is determined chiefly by the rate with which the pellet is heated. When the heating rate is <30 K min −1 , the synthesis process is a solid-state reaction resulting in intermediate products that require temperatures >573 K to transform into Cu 2 Se. In the SHS process, Cu 2 Se is formed directly following the passage of the combustion wave and such synthesis effectively controls the composition and yields homogeneous Cu 2 Se in a time span of few seconds. Microstructure of Cu 2 Se The microstructure of Cu 2 Se following the ultra-fast SHS is examined by FESEM, as shown in Supplementary Fig. 4a,b . Two kinds of typical microstructures are present: a matrix of micron-scale size and a corn-like distributed nanostructure with the size of 5–10 nm. TEM image is shown in Supplementary Fig. 4c and depicts several nanostructural features in the micron-scale matrix, consistent with the FESEM results. High resolution TEM images shown in Supplementary Fig. 4d,e indicate inter-planar spacings of 0.206 nm and 0.336 nm, respectively, corresponding to the (541) and (211) crystal faces of α-Cu 2 Se according to JPDS47-1448. Supplementary Fig. 4e shows that the interface between the nanostructure and the matrix is substantially coherent, which has implications for the charge carrier and phonon transport discussed above. Semi-quantitative EDS results demonstrate that the corn-like nanostructure and the matrix are of similar composition. Cu 2 Se obtained after SHS does not have full density and must be crushed and compacted by using SPS, resulting in ingots of better than 98% theoretical density. The evolution of the microstructure following this brief SPS process is shown in Supplementary Fig. 4g,l . The grain size of the matrix remains at about 1–3 μm. While nanodots are observed on grain faces of the matrix having the size of about 30 nm, high resolution TEM images in Supplementary Fig. 4j,k indicate that at least some of the nanodots have the size of 10 nm and are essentially identical to the nanodots prior to SPS. The interface between the nanostructure and the matrix remains substantially coherent. Elemental distribution maps representing the SHS product and the SHS–SPS bulk are shown in Supplementary Fig. 4f,l , respectively. Thermal stability of Cu 2 Se To test the stability of our Cu 2 Se prepared by SHS–SPS, we have annealed samples at 800 K for 3 weeks under vacuum and re-measured their transport properties. Supplementary Fig. 5 shows XRD patterns of samples prior to annealing and following annealing for periods of 1, 2 and 3 weeks. The phase composition of samples is unchanged regardless of whether annealed or not and for how long. Supplementary Fig. 6a,d shows FESEM images for samples before and after annealing. Again, the microstructure of the samples is unchanged following annealing. The grain size is essentially identical and samples are well-compacted and homogeneous. Supplementary Fig. 7a,d displays the temperature dependence of electrical conductivity, Seebeck coefficient, thermal conductivity and ZT for samples with and without annealing. Within error bars of each measurement, the data are the same. Thus, we conclude that the structural and TE properties of Cu 2 Se prepared by SHS–SPS can survive long-term annealing at least to 800 K and the material serves an excellent p -type semiconductor for intermediate temperature power generation applications. How to cite this article : Su, X. et al. Self-propagating high-temperature synthesis for compound thermoelectrics and new criterion for combustion processing. Nat. Commun. 5:4908 doi: 10.1038/ncomms5908 (2014).